Balanced activity in basal ganglia projection pathways is critical for contraversive movements The basal ganglia, and the striatum in particular, have been implicated in the generation of contraversive movements. The striatum projects to downstream basal ganglia nuclei through two main circuits, originating in striatonigral and striatopallidal neurons, and different models postulate that the two pathways can work in opposition or synergistically. Here we show striatonigral and striatopallidal neurons are concurrently active during spontaneous contraversive movements. Furthermore, we show that unilateral optogenetic inhibition of either or both projection pathways disrupts contraversive movements. Consistently, simultaneous activation of both neuron types produces contraversive movements. Still, we also show that imbalanced activity between the pathways can result in opposing movements being driven by each projection pathway. These data show that balanced activity in both striatal projection pathways is critical for the generation of contraversive movements and highlights that imbalanced activity between the two projection pathways can result in opposing motor output. The control of contraversive movement by each brain hemisphere has been extensively studied in neurological patients [1] , [2] . Single hemisphere lesions of the dorsal striatum abolish contraversive movements and bias towards ipsiversive movements [3] , [4] , [5] , while unilateral stimulation of the dorsal striatum induces contraversive movements [6] , [7] . The striatum projects to downstream nuclei through two main circuits, the so-called direct and indirect pathways, which arise from striatonigral and striatopallidal medium spiny projection neurons [8] . Several models have been proposed postulating how these different basal ganglia pathways could control movement. Some models postulate that these pathways have opposing effects on the output of the basal ganglia [9] , [10] , [11] and movement [12] , [13] , [14] , while others say that co-activation of both pathways is necessary for movement [15] , [16] , [17] , [18] . Recent studies revealed concurrent unilateral activation of both striatonigral and striatopallidal neurons when animals perform contraversive movements in an operant task [16] . However, other studies have shown that lesion [14] , [18] , [19] or stimulation of each cell type can have opposite effects on contraversive movements [12] , [13] . Here we used a fibre-optic-based method and the genetically encoded calcium indicator GCaMP6s to measure the activity of striatonigral and striatopallidal neurons during spontaneous contraversive and ipsiversive movements. Furthermore, we used optogenetics to selectively inhibit (or activate) either or both striatal projection pathways unilaterally, and assess their role in contraversive and ipsiversive movements. We observed that both striatonigral and striatopallidal neurons showed an increase in activity during spontaneous contraversive movements, and that inhibiting either or both striatal pathways unilaterally impaired contraversive movements and biased the animals to perform ipsilateral turns. Furthermore, we observed that simultaneous activation of both striatal projection pathways produced contraversive movements. Finally, we also show that activation or inhibition manipulations that caused a strong imbalance of activity between the striatal projection pathways can result in opposing movements being driven by each pathway. Striatal activity during spontaneous contraversive movements To monitor the activity of the striatonigral and striatopallidal neurons during spontaneous contraversive movements we expressed GCaMP6s specifically in each cell type. We used this by injecting viruses that express GCaMP6s in a Cre-dependent manner (Flex, AAV2/1, see Methods) into the dorsal striatum of mice expressing Cre in either striatonigral ( D1 Cre mice—EY217) or striatopallidal neurons ( A2A Cre mice—KG139) [16] , [20] . To monitor bulk fluorescence of GCaMP during activity of a specific cell population we implanted fibre optics into the dorsal part of the striatum, and coupled these fibres with a detection system using a photomultiplier (PMT) (see methods and Fig. 1a ). After 3–4 weeks (for GCaMP6s to express), we placed animals into a novel arena (a novel cage similar to the home cage) and monitored their behaviour using video and changes in GCaMP6s fluorescence using the system described above ( Fig. 1a ). We used a custom-made software platform (see Methods) to perform online tracking of the body of the animals, and offline analysis to identify spontaneous ipsi or contraversive movements ( Fig. 1c,f ). We observed that both striatonigral and striatopallidal neurons showed an increase in activity during spontaneous contraversive movements (481 trials for contralateral turns from 4 D1-Cre hemispheres infected with GCaMP6s, P <0.05; 2005 trials for contralateral turns of 4 A2A-Cre hemispheres infected with GCaMP6s, P <0.05 from 4 A2A-Cre hemispheres infected with GCaMP6s, P <0.05; Mann–Whitney test; Fig. 1d,g ). Furthermore, to better assess the temporal resolution of the increase in fluorescence, we performed a cross-correlation between the ipsi or contraversive angular velocity and the GCaMP6s signal. We observed that the significant increase in activity of both striatal pathways preceded the changes in angular velocity. Furthermore, we observed a decrease in GCaMP6s fluorescence during ipsiversive movements ( P <0.05 for ipsi or contralateral turns; Fig. 1h : n= 4 hemispheres; Mann–Whitney test). The corresponding controls expressing only eYFP did not show any significant changes in fluorescence during either contra or ipsiversive movements (inserts in Fig. 1d–h : 196 trials for ipsilateral and 283 trials for contralateral turns from 2 D1-Cre hemispheres infected with eYFP ; 1,514 trials for ipsilateral and 1,421 trials for contralateral turns from 2 A2A-Cre hemispheres infected with eYFP ; Mann–Whitney test). 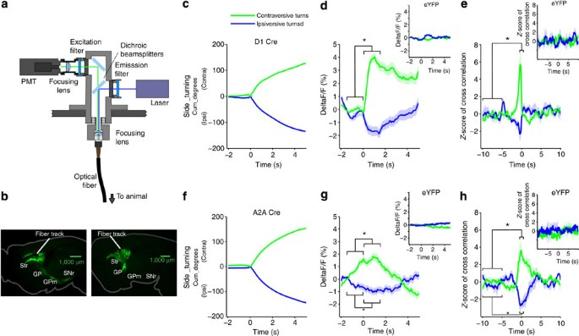Figure 1: Increase activation of the basal ganglia pathways during spontaneous contraversive movements. (a) Schematics of fibre optic setup for acquisition of bulk fluorescence from specific cell populations. (b) GCaMP6s fluorescence in the striatonigral (left) and striatopallidal (right) pathways in brain slices of mice used in the experiments. (c,f) Mean (of all trials of GCaMP6s-infected mice) temporal dynamics of the cumulative degrees of turning over 7 s inD1-CreandA2A-Crelines, aligned to two seconds before the turn, blue: ipsilateral side; green: contralateral side. Data is presented as mean± s.e. (d,g) Mean change in fluorescence (ΔF/F0) of all trials of GCaMP6s infected mice during contra and ipsilateral turns for the two pathways aligned to 2 s before the turn. Insets: mean ΔF/F0foreYFPcontrols. *P<0.05, for a Mann–Whitney test;n=4D1-Creand 4A2A Crehemispheres infected with GCaMP6s. (e,h) Mean (of all hemispheres)Z-score of the cross-correlation between the fluorescence data and the angular velocity, ipsiversive and contraversive, for theD1-CreandA2A-Cremouse lines infected with GCaMP6s. Inset:Z-score of cross-correlation ineYFPcontrols. *P<0.05, for a Mann–Whitney test;n=4D1-Creand 4A2A Crehemispheres infected, same data as fromdandg. Str: striatum; GP: globus pallidus; GPm: medial globus pallidus; SNr: sustantia nigra pars reticulata. Figure 1: Increase activation of the basal ganglia pathways during spontaneous contraversive movements. ( a ) Schematics of fibre optic setup for acquisition of bulk fluorescence from specific cell populations. ( b ) GCaMP6s fluorescence in the striatonigral (left) and striatopallidal (right) pathways in brain slices of mice used in the experiments. ( c , f ) Mean (of all trials of GCaMP6s-infected mice) temporal dynamics of the cumulative degrees of turning over 7 s in D1-Cre and A2A-Cre lines, aligned to two seconds before the turn, blue: ipsilateral side; green: contralateral side. Data is presented as mean± s.e. ( d , g ) Mean change in fluorescence (ΔF/F 0 ) of all trials of GCaMP6s infected mice during contra and ipsilateral turns for the two pathways aligned to 2 s before the turn. Insets: mean Δ F / F 0 for eYFP controls. * P <0.05, for a Mann–Whitney test; n= 4 D1-Cre and 4 A2A Cre hemispheres infected with GCaMP6s. ( e , h ) Mean (of all hemispheres) Z -score of the cross-correlation between the fluorescence data and the angular velocity, ipsiversive and contraversive, for the D1-Cre and A2A-Cre mouse lines infected with GCaMP6s. Inset: Z -score of cross-correlation in eYFP controls. * P <0.05, for a Mann–Whitney test; n= 4 D1-Cre and 4 A2A Cre hemispheres infected, same data as from d and g . Str: striatum; GP: globus pallidus; GPm: medial globus pallidus; SNr: sustantia nigra pars reticulata. Full size image Inhibiting the activity of striatal projection pathways To test whether the observed increase in activity of both projection pathways was necessary for contraversive movements we performed optogenetic inhibition of striatonigral and striatopallidal neurons (either simultaneously or independently) while animals performed spontaneous movements in a small open field. To optogenetically inhibit striatonigral and striatopallidal neurons we expressed Archaeorhodopsin (ArchT-GFP) in a Cre-dependent manner [21] . To achieve simultaneous inhibition of both striatal projection pathways we expressed ArchT in a Cre-dependent manner [20] in RGS9L-Cre mice, which targets both striatonigral and striatopallidal neurons [22] . We injected viruses expressing ArchT-GFP in a Cre-dependent manner (Flex, AAV2/1 (ref. 23 ) into the sensorimotor or dorsolateral striatum of RGS9L-Cre mice, and achieved strong GFP expression in both striatal pathways ( Supplementary Fig. 1a ). We verified that a similar proportion of cells from each striatal projection pathway was infected in RGS9L-Cre mice by crossing RGS9L-Cre animals with either D1-tdTomato or D2-eGFP [20] , [24] , and injecting a Cre-dependent virus expressing the other fluorophore into the dorsolateral striatum of these animals (~50% of the RGS9L Cre cells are either D1 positive or D2 positive, see the anatomical verification Methods). To achieve selective expression of ArchT-GFP in either the striatonigral or the striatopallidal pathways, we injected the same ArchT-GFP virus into the dorsolateral striatum of either D1 Cre mice (EY217) or D2 Cre and A2A cre mice (ER43 and KG139; both lines were used to ensure that the effects observed were specific to the manipulation of striatopallidal pathway neurons, as D2 receptors may be expressed in different striatal interneurons [13] , Supplementary Fig. 1a,b ). Using stereological counting, we determined that we infected on average 32.5% of striatal cells in the infected area in RGS9L-Cre mice (peak infection area ~58%), 26.5% in D1 and 31.5–32.5% in D2 and A2A Cre mice (peak infection area 45–50%, respectively). Furthermore, we verified ex vivo and in vivo that green light illumination did cause inhibition of firing in ArchT-GFP- expressing neurons (556 nm, 9.2±1.2 mW × mm −2 was the minimum power to decrease spiking of striatal cells in the slice; in vivo we used 25–35 mW measured at the fibre tip to achieve a wider modulation, 57 ms was the average latency to inhibit firing in vivo , Fig. 2 ). 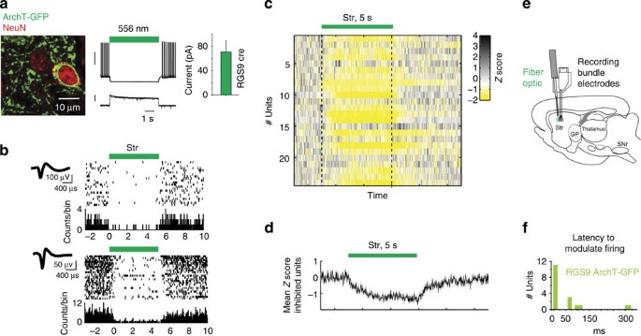Figure 2: Inhibition of striatal neurons during unilateral ArchT stimulation and ipsiversive turns. (a) Left panel, photomicrograph from a cell expressing ArchT and positive for inmunolabelling the nuclei using NeuN (cumulative intensity from four frames taken every 1 μm). Right panel, voltage and current responses to green light illumination in a striatal projection neuron recorded in a brain slice, the bar on the right panel shows the mean current in response to 9.2 mW × mm−2(minimum power to inhibit spikes in striatal neurons), upper and lower vertical bars: 30 mV and 50 pA, respectively. (b) Peri-event histograms examples from individual units aligned to the onset of green light stimulation presented inc, bottom to top trials. (c) Peri-event histograms of theZ-scored timestamps of extracellularly recorded action potentials of striatal neurons in the ipsilateral side, aligned to the onset of light in freely moving mice expressing ArchT-GFP, while turning ipsilateraly in an open field. Timestamps of each spike for the different cells, aligned to the onset of green light illumination. (d) MeanZ-score for the units that were significantly modulated by the green light stimulation. (e) Representative diagram illustrating the recordings and light stimulation inside the striatum of animals treated to express ArchT. (f) Latency to modulate spikes in ArchT-expressing striatal cells. Figure 2: Inhibition of striatal neurons during unilateral ArchT stimulation and ipsiversive turns. ( a ) Left panel, photomicrograph from a cell expressing ArchT and positive for inmunolabelling the nuclei using NeuN (cumulative intensity from four frames taken every 1 μm). Right panel, voltage and current responses to green light illumination in a striatal projection neuron recorded in a brain slice, the bar on the right panel shows the mean current in response to 9.2 mW × mm −2 (minimum power to inhibit spikes in striatal neurons), upper and lower vertical bars: 30 mV and 50 pA, respectively. ( b ) Peri-event histograms examples from individual units aligned to the onset of green light stimulation presented in c , bottom to top trials. ( c ) Peri-event histograms of the Z -scored timestamps of extracellularly recorded action potentials of striatal neurons in the ipsilateral side, aligned to the onset of light in freely moving mice expressing ArchT-GFP, while turning ipsilateraly in an open field. Timestamps of each spike for the different cells, aligned to the onset of green light illumination. ( d ) Mean Z -score for the units that were significantly modulated by the green light stimulation. ( e ) Representative diagram illustrating the recordings and light stimulation inside the striatum of animals treated to express ArchT. ( f ) Latency to modulate spikes in ArchT-expressing striatal cells. Full size image Inhibiting either pathway favours ipsiversive movements We inhibited either or both striatal pathways unilaterally by delivering green light into the dorsolateral striatum through an optical fibre ( Supplementary Fig. 1 ) on either hemisphere in the same mouse (5 s of continuous light delivery per stimulation, ~67 s time between stimulations (mean interval: 67±9 s, max: 500, min: 21 s—and mean number of trials per animal of 9, max: 20, min: 3)), and evaluated contraversive versus ipsiversive locomotion in freely moving mice in an open field (using a custom-made software to analyse deviations from the rostrocaudal axis, see Methods). Assuming a cone of light emanating from the 0.48-numerical aperture (NA) fibre, and considering the minimum power intensity to modulate the spiking of striatal and the mean average of cells expressing the opsin (~30%), we estimated to be manipulating ~4,601–5,813 neurons per striatum (see Methods). We observed that inhibiting either or both striatal pathways unilaterally for 5 s impaired contraversive movements and biased the animals to perform ipsilateral turns ( Fig. 3 ). We first tested whether selective inhibition of either striatonigral and striatopallidal neurons would decrease contraversive turns and bias the animals to turn ipsilaterally. We verified that inhibiting the striatonigral neurons unilaterally resulted in ipsilateral turning (both group and interaction effects when compared with D1-eYFP controls; F time =13.21; F group =4.27; F interaction time × group =1.64; P <0.05; repeated measures analysis of variance, Fig. 3a–c ). Inhibition of striatonigral neurons in the right striatum resulted in turning towards the right side of the animal, while inhibition of striatonigral neurons in the left striatum resulted in turning towards the left ( Fig. 3a–c , D1-ArchT Lside-Inhibition : 45±10 cumulative degrees to the left versus D1-ArchT Rside-Inhibition : −39±7 cumulative degrees to the right; n= 9, within-subject comparison against baseline before stimulation, and also between left and right for each mouse; post-hoc Wilcoxon test, P <0.05). A similar effect was observed with unilateral inhibition of striatopallidal neurons (both group and interaction effects when compared with eYFP controls, F time =14.54; F group =7.18; F interaction time × group =5.64; P <0.05; Fig. 3d–f D2/A2A-ArchT Lside-inhibition : 59±29 versus D2/A2A-ArchT Rside-inhibition : −86±25, Wilcoxon test, P <0.05, n= 10; Wilcoxon test, P <0.05 against baseline and also left versus right stimulation). This was not observed if light was delivered into D1-Cre or A2A/D2-Cre animals carrying a control Cre-dependent eYFP virus ( D1-Cre eYFP , n= 8, and A2A/D2-Cre eYFP , n= 6, Wilcoxon test, P >0.05 against baseline and also left versus right stimulation; n= 6, D2/A2A ArchT versus D2/A2A eYFP , Kruskal–Wallis, P <0.05 Fig. 1h ; D1-ArchT versus D1-eYFP , P >0.05). 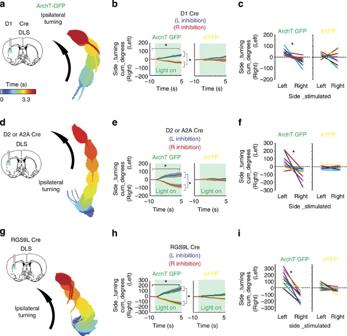Figure 3: Simultaneous or independent inhibition of each striatal pathway biases towards ipsiversive movements. (a,d,g) Representative time series of video frames during the 5 s of unilateral left inhibition of the striatonigral, striatopallidal and both pathways, respectively (colours from blue to red show evolution of the behaviour during the stimulation period). (b,e,h) Temporal dynamics of the cumulative degrees of turning over the 5 s of stimulation in response to unilateral inhibition of striatal cells in the different Cre lines, aligned to one second before the illumination, blue: left side inhibition; red: right side inhibition. Data is presented as mean±s.e. (c,f,i) Average cumulative degrees of turning towards left or right side, per animal, during the last second of unilateral inhibition, the striatonigral pathway alone, the striatopallidal pathway alone and both striatal pathways simultaneously. *P<0.05, for a within-animal Wilcoxon test;n=9 andn=10 for D1 and D2/A2A CreArchT GFP;n=8 andn=6 for D1 and D2/A2A Cre eYFP.D1 Cre: line targeting the striatonigral pathway. D2/A2ACre: lines targeting the striatopallidal pathway and RGS9LCre: line targeting simultaneously both the striatonigral and the striatopallidal pathway simultaneously. Figure 3: Simultaneous or independent inhibition of each striatal pathway biases towards ipsiversive movements. ( a , d , g ) Representative time series of video frames during the 5 s of unilateral left inhibition of the striatonigral, striatopallidal and both pathways, respectively (colours from blue to red show evolution of the behaviour during the stimulation period). ( b , e , h ) Temporal dynamics of the cumulative degrees of turning over the 5 s of stimulation in response to unilateral inhibition of striatal cells in the different Cre lines, aligned to one second before the illumination, blue: left side inhibition; red: right side inhibition. Data is presented as mean±s.e. ( c , f , i ) Average cumulative degrees of turning towards left or right side, per animal, during the last second of unilateral inhibition, the striatonigral pathway alone, the striatopallidal pathway alone and both striatal pathways simultaneously. * P <0.05, for a within-animal Wilcoxon test; n= 9 and n= 10 for D1 and D2/ A2A Cre ArchT GFP; n= 8 and n= 6 for D1 and D2/ A2A Cre eYFP . D1 Cre : line targeting the striatonigral pathway. D2/A2ACre: lines targeting the striatopallidal pathway and RGS9LCre: line targeting simultaneously both the striatonigral and the striatopallidal pathway simultaneously. Full size image Furthermore, simultaneous inhibition of both striatonigral and striatopallidal neurons unilaterally resulted in ipsiversive turning (both group and interaction effects when compared with RGS9L-eYFP controls, F time =42.48; F group =17.7 F interaction time × group =16.22; P <0.05; repeated measures analysis of variance). Inhibition of both striatal projection pathways in the right striatum resulted in turning towards the right side of the animal, while inhibition of both cell types in the left striatum resulted in turning towards the left ( RGS9L-ArchT Lside-inhibition : 137±35, cumulative degrees to the left, and RGS9L-ArchT Rside-inhibition : −115±27, cumulative degrees to the right; n= 9, P <0.05, within-subject comparison against baseline before stimulation, and also between left and right for each mouse; Wilcoxon test, Fig. 3g–i ). This was not observed if light was delivered into RGS9L-Cre animals carrying a Cre-dependent eYFP virus ( n= 9, P >0.05, Fig. 1j,k : RGS9L-ArchT GFP versus RGS9L-eYFP , Kruskal–Wallis, P <0.05; Fig. 3h ). Taken together, these results indicate that activity in either the striatonigral or the striatopallidal pathways is required for contraversive movements. Interestingly, the additive effect of inhibiting either striatonigral or striatopallidal neurons independently was equivalent to the effect of modulating simultaneously both striatal pathways ( D1-ArchT : 43±8 and D2/A2A-ArchT : 73±19 versus RGS9L-ArchT : 138 ±22; cumulative degrees relative to the side of stimulation), suggesting that activity in both projection pathways contributes to contraversive movements. Inhibiting either pathway impairs contraversive movements The data presented above show that inhibition of either or both striatal projection pathways biases animals towards ipsilateral turns, but does not distinguish if inhibition of the striatal pathways impedes contralateral turns or further favours ipsilateral turns. Therefore, we performed analyses wherein we examined separately trials where animals were turning ipsilaterally or contralaterally just before the onset of inhibition (analysing ~200 ms before inhibition). These analyses allowed us to examine separately optogenetic trials in which both striatonigral and striatopallidal neurons show increased activity (contralateral turning) versus trials where they are not activated and even display a decrease in activity (ipsilateral turns) ( Fig. 4 ). We observed that the specific inhibition of striatonigral neurons impaired contralateral turns (when compared with trials with light off—no inhibition, D1 Cre ArchT-contra off light: −5±4 cumulative degrees to the contralateral side, n= 69 trials versus D1 Cre ArchT-contra on light : 11±4 cumulative degrees to the ipsilateral side, n= 84 trials, Kruskal–Wallis, P <0.05; Fig. 4a,b ), but did not affect ipsilateral turns (again compared with trials with light off—no inhibition, D1 Cre ArchT-ipsi off light : 7±4 cumulative degrees to the ipsilateral side, n= 69 trials, versus D1 Cre ArchT-ipsi on light : 12±5 cumulative degrees to the ipsilateral side, n= 84 trials, Kruskal–Wallis, P >0.05; Fig. 4a,b ). Similarly, inhibition of striatopallidal neurons decreased contralateral turns ( D2 Cre ArchT-contra off light : −5±5 cumulative degrees to the contralateral side, n= 81 trials, versus D2 Cre ArchT-contra on light : 18±5 cumulative degrees to the ipsilateral side, n= 89 trials, Kruskal–Wallis, P <0.05, Fig. 2c,d ), but had no effect on ipsilateral turns ( D2 Cre ArchT-ipsi off light , 10±5 cumulative degrees to the ipsilateral side, n= 81 trials, versus D2 Cre ArchT-ipsi on light , 17±6 cumulative degrees to the ipsilateral side, n= 89 trials, Kruskal–Wallis, P >0.05, Fig. 4c,d ). These data show that inhibition of either striatonigral and striatopallidal neurons impedes contralateral turns (when neurons from both pathways are activated) but did not further bias ipsilateral turns (when neurons from both pathways are not activated and even decrease activity), indicating that activity of each projection pathway is necessary for contralateral turning, but inhibition of an individual pathway is not sufficient to bias further ipsilateral turns. 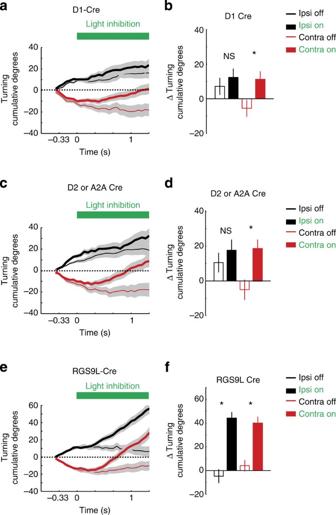Figure 4: Effect of ArchT inhibition on contraversive versus ipsiversive movements. (a,c,e) Mean±s.e. of the individual trials from all animals categorized as ipsilateral turning (black colour) and contralateral turning (red colour) 200 ms before the onset of light, grey shadows represent thes.e. The thick lines correspond to trials receiving light illumination as depicted by the green bar on top of each panel, while the thin lines corresponds to similar segments of time with no light illumination (obtained from periods of 6 s before light onset). (b,d,f) Difference between cumulative degrees at the onset of light (0 s) and 1.33 s after light onset (20 frames later). Figure 4: Effect of ArchT inhibition on contraversive versus ipsiversive movements. ( a , c , e ) Mean±s.e. of the individual trials from all animals categorized as ipsilateral turning (black colour) and contralateral turning (red colour) 200 ms before the onset of light, grey shadows represent thes.e. The thick lines correspond to trials receiving light illumination as depicted by the green bar on top of each panel, while the thin lines corresponds to similar segments of time with no light illumination (obtained from periods of 6 s before light onset). ( b , d , f ) Difference between cumulative degrees at the onset of light (0 s) and 1.33 s after light onset (20 frames later). Full size image We next examined the effect of inhibiting both striatonigral and striatopallidal neurons simultaneously. Inhibition of both projection pathways impeded contralateral rotations and further biased ipsilateral rotations ( RGS9L Cre ArchT-ipsi off light : −4±5 cumulative degrees to the ipsilateral side, n= 86 trials, versus RGS9L Cre ArchT-ipsi on light : 43±5 cumulative degrees to the ipsilateral side, n= 100 trials, Kruskal–Wallis, P >0.05. RGS9L Cre ArchT-contra off light : 4±4 cumulative degrees to the ipsilateral side, n= 105 trials, versus RGS9L Cre ArchT-contra on light : 39±5 cumulative degrees to the ipsilateral side, n= 92 trials, Kruskal–Wallis, P >0.05, Fig. 4e,f ). These data show that activity in either striatonigral or striatopallidal neurons is necessary for contralateral turns, but inhibition of an individual cell type is not sufficient to further bias ipsilateral turns; only when both striatonigral and striatopallidal neurons are simultaneously inhibited unilaterally can ipsilateral turns be further biased (consistent with Fig. 1 and with ref. 16 ). Striatal activity biases head movements The results presented so far suggest that although we only manipulate a few thousand neurons in sensorimotor striatum, this affects whole body movements. However, as our optogenetic manipulations were targeting areas in the striatum receiving input from head areas of motor cortex [25] we decided to investigate whether our manipulations affected contraversive movements of the head in relation to the body axis. To assess contraversive and ipsiversive movements of the head in relation to the longitudinal body axis during stimulation we analysed angle of the head and of the body independently (and subtracted whole body turning, see Methods and Fig. 5a ). These analyses revealed that inhibition of both striatonigral and striatopallidal neurons produced ipsiversive head movements (comparing 1 s before light onset versus a 1-s sliding window after inhibition; Kruskal–Wallis, P <0.05, Fig. 5b ). To distinguish whether inhibition of the striatal projection pathways impedes contralateral turns or further favours ipsiversive movements of the head, we analysed the effect of manipulating the striatal activity in trials in which the head was turning contraversively versus trials in which the head was turning ispiversively before the onset of inhibition (200 ms). We observed that inhibition of both striatonigral and striatopallidal neurons impeded contraversive head movements, but did not further bias ongoing ipsiversive head movements (Kruskal–Wallis, P <0.05, Fig. 5c , brackets to the right; after verifying overall effect, post-hoc analyses frame by frame revealed the specific period of time showing significant decrease in contraversive movements, horizontal bracket in Fig. 5c corresponding to the bars presented in Fig. 5d ). 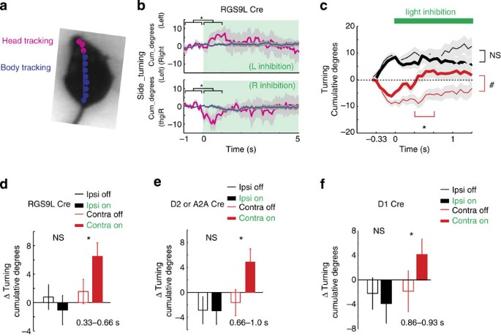Figure 5: Contraversive and ipsiversive movements of the head in relation to the body. (a) Representative example of the animal segmentation separating the head tracking (magenta) from body tracking (dark blue; see methods). (b) Temporal dynamics of the cumulative degrees of head turning towards each side during the 5 s of unilateral illumination to inhibit both striatal pathways (shadowed green and blue square), magenta: head tracking, dark blue: body tracking. (c) Mean±s.e. of the individual trials from all animals categorized as ipsilateral head turning (black colour) and contralateral head turning (red colour) 200 ms before the onset of light, grey shadows represent the s.e. The thick lines correspond to trials receiving light illumination as depicted by the green bar on top of each panel, while the thin lines corresponds to turns in the same animals with no light illumination (obtained from periods of 6 s before light onset). (d) Difference between cumulative degrees at the onset of light (0 s) and the time depicted by the horizontal brackets inc. (e) Same analyses as forcandd, in this case for inhibition the striatopallidal pathways. (f) Same analyses as forcandd, in this case for inhibition of the striatonigral pathways. #P<0.05, Kruskall–Wallis, for the total period of illuminations. *P<0.05 for thepost hocsin the period of time depicted by the horizontal bracket. The inserted periods of time correspond to the periods of time in which theposthocanalysis showed significance. Figure 5: Contraversive and ipsiversive movements of the head in relation to the body. ( a ) Representative example of the animal segmentation separating the head tracking (magenta) from body tracking (dark blue; see methods). ( b ) Temporal dynamics of the cumulative degrees of head turning towards each side during the 5 s of unilateral illumination to inhibit both striatal pathways (shadowed green and blue square), magenta: head tracking, dark blue: body tracking. ( c ) Mean±s.e. of the individual trials from all animals categorized as ipsilateral head turning (black colour) and contralateral head turning (red colour) 200 ms before the onset of light, grey shadows represent the s.e. The thick lines correspond to trials receiving light illumination as depicted by the green bar on top of each panel, while the thin lines corresponds to turns in the same animals with no light illumination (obtained from periods of 6 s before light onset). ( d ) Difference between cumulative degrees at the onset of light (0 s) and the time depicted by the horizontal brackets in c . ( e ) Same analyses as for c and d , in this case for inhibition the striatopallidal pathways. ( f ) Same analyses as for c and d , in this case for inhibition of the striatonigral pathways. # P <0.05, Kruskall–Wallis, for the total period of illuminations. * P <0.05 for the post hocs in the period of time depicted by the horizontal bracket. The inserted periods of time correspond to the periods of time in which the posthoc analysis showed significance. Full size image Imbalanced activity between the pathways causes opposing effects In the results presented above we have described ipsilateral biases when inhibiting either of the basal ganglia pathways. This is consistent with the idea that the increased activity of the two pathways during contralateral turning is critical for the foretold movements. However, there is evidence suggesting that independent activation of striatonigral and striatopallidal neurons [12] , [13] or lesions/decreases in the activity of these neurons [18] , [19] leads to opposite effects on behaviour. One discrepancy between these studies and our study could be that either independent activation of each projection pathway or large lesions of one of the cell types would lead to an imbalance in the activity of both pathways, and this could result in opposing behavioural phenotypes. We therefore examined the effect of independently increasing the activity of striatonigral and striatopallidal neurons. We expressed ChR2-eYFP in striatonigral and striatopallidal neurons [12] , [13] , using the same strategy used for expressing ArchT ( Supplementary Fig. 1 ), and stimulated each striatum of each mouse for 5 s (we used 10 ms pulses delivered at 14 Hz, ~44 s inter-trial interval when using more that a single trial—44±4 s (max: 175, min: 14 s), number of trials when using more than a single stimulation, mean: 3 (min: 2, max: 12 trials)). As previously shown [12] , [13] , selective stimulation of striatonigral neurons favoured contralateral movements, while selective stimulation of striatopallidal neurons resulted in ipsilateral turns ( Supplementary Fig. 2b,e ). However, if both pathways are simultaneously activated, as observed when monitoring their activity during contralateral turns ( Fig. 1 ), animals perform contralateral movements ( RGS9L-ChR2 Lside-activation : −187±28 cumulative degrees to the left and RGS9L-ChR2 Rside-activation : 192±45 cumulative degrees to the right; Wilcoxon test, P <0.05, against baseline and left versus right; n= 6, Supplementary Fig. 3 ; no effect in eYFP controls). These data suggest that although simultaneous activity of both pathways is normally involved in contralateral turns, imbalanced activity between the two projection pathways can lead to opposite effects in movement, which could be relevant for some disorders. To further investigate this we also performed more extensive inhibition of each striatal projection pathway ( Supplementary Fig. 2k–t ) by crossing D1 Cre or A2A Cre animals with the Ai35 mouse line (expressing ArchT in all Cre-positive cells [26] ). We observed that unilateral striatal inhibition on the dorsolateral part of the striatum in the D1-Cre Ai35 animals induced ipsiversive movements ( Supplementary Fig. 2l ), whereas inhibition of the dorsolateral part of the striatum in A2A Cre Ai35 animals induced contraversive movements ( Supplementary Fig. 2o ), consistent with refs 18 , 19 . The results presented above suggest a more complex functional organization of basal ganglia circuits than initially thought. Therefore, we performed electrophysiological recordings of neural activity in striatum and downstream target regions (globus pallidus, substantia nigra reticulata (SNr) and primary motor cortex) to investigate whether the effects in downstream neurons were those predicted ( Supplementary Fig. 4 ). Although ArchT stimulation caused strong inhibition of striatonigral and striatopallidal projection neurons ( Supplementary Fig. 4a-d ), the classically predicted opposing effects in basal ganglia output (SNr) were not observed ( Supplementary Fig. 4e–g ). Inhibition of striatonigral neurons did not lead to an increase in activity in SNr (few neurons changed activity and a similar proportion of neurons increased versus decreased activity), whereas inhibition of striatopallidal neurons did result in an increase in activity in GPe, but not in a decrease of activity in SNr ( Supplementary Fig. 4g ). Together with the effects observed in the primary motor cortex, these results suggest the existence of functional connectivity details in basal ganglia circuitry that are beyond the known feedforward connections classically reported [27] , [28] , [29] . The findings presented here suggest that co-activation of striatonigral and striatopallidal neurons is critical for natural contraversive movements. Using a new method of photometry through fibre optics to measure GCaMP6s activation, we observed that striatonigral and striatopallidal neurons are concurrently active during spontaneous contraversive movements, and slightly decrease activity during ipsilateral turns ( Fig. 1 ; consistent with ref. 16 ). These measurements reflect the bulk activity of thousands of neurons [16] , and so they probably represent the population average of the activity of striatonigral and striatopallidal neurons (which are similar in number) during contraversive movements. However, the spatial resolution of bulk activity and the temporal resolution of GCaMP6s activation are not amenable to differentiate the activity of subpopulations of neurons, or to examine small differences in the time course of activation of both populations [30] . Consistent with the findings that both projection pathways are active during contraversive movements, we showed that optogenetic unilateral inhibition of either striatal projection pathway impaired contralateral movements without affecting ipsilateral movements. Inhibition of both pathways cancelled contralateral turns and further biased ipsilateral turns. These findings support a view in which activity in both projection pathways is required to achieve a particular movement [15] , [16] , [17] , where, for example, direct pathway neurons could select the desired motor programme while indirect pathway neurons inhibit competing motor programmes [16] , [17] , [30] , [31] . This view is further supported by the fact that concurrent activation of direct and indirect pathways caused contralateral turns. Analyses of contraversive and ipsiversive movements of the head in relation to the body axis further confirmed these findings. Still, we also show that imbalance in activity of striatonigral versus striatopallidal neurons can cause opposing motor phenotypes [9] , [10] , [11] , [12] , [13] . This could be at play in disorders in which one of the pathways is strongly activated relative to the other, as suggested, for example, for Parkinson’s and Huntington’s disease [10] , [32] . Furthermore, we verified that inhibiting striatonigral versus striatopallidal neurons does not produce the predicted effects in basal ganglia output. Taken together, these results suggest that the functional connectivity in basal ganglia is more complex than previously thought. For example, the observation that striatopallidal activation in the absence of simultaneous striatonigral activation leads to ipsiversive movements, but in the presence of simultaneous striatonigral activation leads to contraversive movements is intriguing. One potential explanation for the apparent discrepancy is that striatopallidal neuron activation could cause inhibition of striatonigral neurons via the collaterals between them [33] (which are stronger than the converse case [34] ). However, other possibilities that do not rely only on intrastriatal interactions between the pathways are likely to be at play. For example, it is possible that striatonigral versus striatopallidal neurons project to overlapping but not completely redundant downstream target areas of basal ganglia output, so that overactivation or overinhibition of each projection pathway by itself would lead to a different pattern of activation or inhibition of downstream targets than concurrent activation of both pathways. It is also likely to be, given that the main discrepancies were observed after striatopallidal manipulations, that striatopallidal neurons connect to more targets than those postulated by the ‘indirect pathway’, and that pallidal neurons projecting to regions other than the subthalamic neurons and SNr are mediating some of the effects observed here. In conclusion, these data suggest that striatal projection pathways interact to produce desired movements, and that balanced activity in both types of projection neurons is required to produce contraversive movements. Imbalanced activity between the two pathways can lead to opposite motor output. Animals All procedures were reviewed and performed in accordance with the Instituto Gulbenkian de Ciência and the Champalimaud Centre for the Unknown Ethics Committee guidelines, and approved by the Portuguese Veterinary General Board (Direcção Geral de Veterinária, approval ID 018831). Male mice between 2 and 4 months of age, resulting from the backcrossing of BAC transgenic mice into Black C57BL for at least six generations (which express the Cre recombinase under the control of the dopamine D1a (EY217 line), D2 (ER43 line) or A2A (K139 line), or td-tomato or enhanced green fluorescent protein, under the promoters of D1 or D2 receptors obtained from GENSAT [20] ) into C57BL/6J (The Jackson Laboratory) were used in this study. Stereotaxic virus injections and fibre implantation Surgeries were performed under deep anaesthesia using a mix of oxygen (1 l min −1 ) and 1% isuoflorane (1–3% for interventional procedures). For GCaMP6s experiments, animals were infected and implanted either in only one hemisphere or in both. In each hemisphere, 1 μl of viral stock solution was injected using quartz pipettes and a picospritzer (Parker Hannifin) in the dorsal striatum at coordinates anteroposterior 0.5 mm from the bregma, 1.7 mm mediolateral, 2.2 mm deep for D1-Cre mice, and anteroposterior 0.5 mm from the bregma, 2.0 mm mediolateral, 2.45 mm deep for D2-Cre mice. For optogenetic manipulation experiments, each animal was bilaterally injected, using glass pipettes (<50 μm tip), with 1 μl viral stock solution (from a 4- to 5-μl viral aliquot kept at −80 °C) by pressure (4.6 nl every 5 s; 23 nl s −1 rate) using a nonoject II (Drummond Scientific) into the dorsolateral striatum at the following coordinates: anteroposterior: 0.5 mm from the bregma, mediolateral: 2.3 mm and depth: 2.3 mm below the surface of the brain. After the injection was performed, the pipette was left in place for 10 min before retraction. Subsequently, a 200-μm diameter (NA 0.22 for ChR2) or 300-μm diameter (NA 0.48 for ArchT) or 300-μm diameter (NA 0.22 for GCaMP6s) fibre optics were implanted (Doric Lenses) 200-μm above the viral injection. These experiments were carried out using AAV1.Syn.Flex.GCaMP6s (titre 2.98 × 10 13 , University of Pennsylvania), AAV1.EF1a.DIO.ChR2-eYFP (titre 1.4 × 10 13 ; University of North Carolina), AVV1.EF1a.DIO.eYFP (titre 1.4 × 10 13 , University of North Carolina), AVV1.EF1a.Flex.ArchT-GFP (titre 1.4 × 10 12 , University of Pennsylvania) or AVV1.EF1aDIO.td- tomato (titre 1.4 × 10 12 , University of Pennsylvania). Monitoring activity with GCaMP6s The bulk fluorescence acquisition setup consisted of a 473-nm diode-pumped solid-state laser (Crystalaser) for excitation of the fluorophore, which was attenuated with absorptive neutral density filters (Thorlabs), an excitation filter (473 nm Semroc) and two dichroic mirrors for separation of wavelengths (Chroma T495LP and Semrock FF552-DiO2-25 × 36), a focusing lens for the laser beam ( F =12 mm, Doric Lenses), an emission filter (Chroma ET525/50m) and a focusing lens ( F =40 mm, Thorlabs) before the photodetector. To deliver the excitation light to the brain-infected area and to collect the emitted light, a single multimode silica optical fibre with 300 μm core and 0.22 NA was used (Doric Lenses). Light power at the tip of this patchcord fibre was 200 μW for all GCaMP6s experiments (measured before each experiment with a powermeter (PM130D, Thorlabs). The photodetector was a photomultiplier tube module (H7422-02, Hamamatsu Photonics). The control and acquisition of the Transistor–transistor logic (TTL) signal used for synchronization with the video through an light-emitting diode (LED) and the acquisition of the fluorescence signal were performed with an NI-PCI data acquisition board (PCI-6229) at 1 kHz and custom software programmed in Matlab (MathWorks, MA). Two to four weeks after surgery the animals were placed into a novel arena (a novel cage similar to the home cage) while connected to the bulk fluorescence acquisition setup through the optical fibre. Video recordings were done using a PS3 camera (PlayStation) at 60 frames per second and online tracking was done using a custom data processing stream programmed in Bonsai ( https://bitbucket.org/horizongir/bonsai ). Tracking data (angle or angular velocity) and fluorescence data were low-pass filtered at 5 Hz and used for further analysis. Turns were detected by finding the points at which the derivative of the angle was zero and were classified as right or left, depending on whether this derivative was increasing or decreasing, respectively. Only those turns occurring after 5 s in which the s.d. of the angle was smaller than 40° and that after 5 s resulted in a change bigger than 40° were included. Relative changes in fluorescence, Δ F / F 0 =( F − F 0 )/ F 0 was calculated by, for each session, correcting baseline drift with a third-order polynomial. We defined F 0 as the 10th percentile of the drift-corrected fluorescence. All angle and all Δ F / F 0 (subsampled to match the angle data) values during the detected turns were collected in all the sessions of all the mice, separated in contra and ipsilateral sides, and averaged. For easier comparison of contra and ipsilateral Δ F / F 0 traces, each was subtracted by its mean between −2 and −1 s before the turn. For cross-correlation analysis angular velocity was derived from the body angle data, low-pass filtered at 5 Hz and separated into contra- and ipsilateral angular velocity by separating the positive and the negative components of the signal and rectifying them. Filtered and subsampled Δ F / F 0 data and rectified angular velocity data of all sessions of each mouse were concatenated and the cross-correlation of the z -score of the two signals was determined for each mouse. Light manipulations ex vivo Striatal brain slices were obtained as described inref. [33] . In the case of the ChR2-eYFP versus eYFP comparison in vitro , optical stimuli was delivered from 200 μm multimode optical fibres coupled to a 50-mW, 473 nm, diode-pumped, solid-state laser (Laserglow Technologies) or using a fibre-coupled LED (473 nm, Doric Lenses). In the case of the ArchT-GFP versus eYFP experiments, a 200-μm fibre core, 0.48 NA, coupled to a diode-pumped, solid-state laser (CNI Lasers, Changchun, China) was used and the control of delivering the light was done using a shutter (Thorlabs). In all the recordings, the tip of the fibre was positioned 200–400 μm away from the recorded cells. No significant changes on the intrinsic properties of the cells were found when comparing Cre ChR2-eYFP versus Cre eYFP -expressing cells or Cre ArchT GFP versus Cre eYFP- expressing cells, in periods of expression <3 weeks (see Supplementary Fig. 1 ). The minimum power to trigger reliable spikes using ChR2 in vitro was calculated as 1.6 mW × mm −2 . In the case of ArchT we estimated an average current of 71±17 pA in response to 9.2±1.2 mW × mm −2 as the minimum power needed to affect the firing of striatal cell (see Supplementary Fig. 2 ). Light manipulations in vivo For the ChR2 and the corresponding controls, optical stimuli were delivered from 200 μm implantable fibres (NA 0.22; Doric Lenses) coupled to a 200-mW, 473-nm, diode-pumped, solid-state laser (Laserglow Technologies) using a one-input two-outputs rotatory joint (Doric Lenses) clamped in the position that during the day of the experiment was found to deliver the same amount of light on the two outputs. To set up the parameters of ChR2 stimulation we tried different protocols with 5 Hz, 14 Hz or 5 s of continuous light delivery. Although both 5 and 14 Hz provided reliable stimulation, continuous light resulted in an initial activation that was not sustained and rapidly decreased. For the ArchT and the corresponding controls, optical stimuli were delivered using 200 or 300, implantable fibres (NA 0.48; Doric Lenses) free launched to a 500-mW, 556-nm, diode-pumped, solid-state laser (CNI Lasers) using a fibre optic to get light into a one-input two-outputs rotatory joint as for the blue laser. For the blue laser, the delivery of the light was controlled via TTL pulses connected to the diode-pumped solid-state lasers (DPSSL) driver of the laser. All the experiments using ArchT were done using an acoustic optic modulator (AA Opto Electronic) to control the path of the light. Measures of the power in the tip of the fibre (similar to the one implanted) were verified every day of the experiment using a powermeter (PD1000-S130C, Thorlabs) and the power adjusted at the tip of the fibre to be 1–3 mW for ChR2 or 25–35 mW for ArchT, unless otherwise stated. Neuronal recording and light stimulation in vivo To verify and decide the parameters of stimulation we recorded the activity of striatal neurons while delivering light stimulation in freely moving animals in the open field (39 × 39 cm; see Supplementary Fig. 2 ). These animals were previously infected to express either ChR2-eYFP or ArchT-GFP , and implanted with electrode arrays coupled to an implantable fibre. We use two kinds of array-fibre configurations. One of these array configuration consisted of a 2 × 8 array of platinum-coated tungsten microwire electrodes of 35 μm diameter with 150 μm spacing between microwires, and 250 μm spacing between rows coupled to an optic fibre. The second system was a movable bundle of 16 platinum-coated tungsten microwires, which allowed us to record from different distances related to the tip of the fibre (Innovative-Neurophysiology). In both cases these array-fibre configurations contained guide cannulas to introduce a fibre optic positioning it 200–300 μm away from the tip of the electrodes before implantation. The neural activity and the timestamps from the light stimulation were recorded using the Cerebrus recording system (Blackrock Microsystems). The spike activity was initially sorted using an online sorting algorithm (Central Software, Blackrock Microsystems), and only cells with a clearly identified waveform and relatively high signal-to-noise ratio (>3:1) were used for further analyses. At the end of recording, cells were resorted using an offline sorting algorithm (Offline Sorter, Plexon Inc.) to isolate single units and together with the timestamps of the light stimulation provided by a pulse generator (Master 8, AMPI) were exported to MATLAB to perform analyses (see Supplementary Fig. 2 ). To determine the volume of ArchT-positive neurons that can be effectively photostimulated to induce inhibition of spikes in neurons, we estimated the brain volume in which the light intensity achieved is greater than ~9.2 mW × mm −2 (threshold determined as the minimum intensity to modulate the spiking of striatal cells recorded in the slice). From experimental data measuring the light through striatal tissue we estimated that after passing through 100 μm of striatal tissue, total transmitted light power was reduced by 50%, and by 90% at 1 mm ( Supplementary Fig. 1c,f ). The data was fit by a Kubelka–Munk model for diffuse scattering media [35] , with best-fit values for the scattering coefficient of 12.0 and 9.0 mm −1 for 473 nm and 561 light in the striatal mouse tissue. In addition to loss of light from scattering and absorption, light intensity also decreases as a result of the conical spreading of light after it exits the optical fibre. The light exiting the multimode fibre is not collimated and spreads with a conical angle of 41° determined by the numerical aperture of 0.48 used in the case of ArchT and 18° as determined by the numerical aperture of 0.22 used for ChR2. This effect will reduce the light intensity, which is expected to be the relevant quantitative parameter determining efficacy of ArchT or ChR2 stimulation. We therefore calculated the effective intensity, taking into account the combined effects of scattering, absorption and conical spread ( Supplementary Fig. 1d,g ). These calculations allowed us to estimate the expected volume of tissue to modulate the ArchT- or the ChR2-expressing cells by the light illumination in vivo . If effective inhibition of spikes is achieved at 9.2 mW × mm −2 , in principle we were able to inhibit the spikes in 30% of the neurons (average rate of infection) at least up to 0.5 mm from the fibre tip ( Supplementary Fig. 1d ). This distance value, together with the measured conical cross-section of 1.0 and 1.1 mm diameter at 0.5 mm from the fibre tip, results in a total volume experiencing 9.2 mW × mm −2 light intensity of ~0.172–0.217 mm 3 (using 200 and 300 fibre core). Considering this volume and taking into account that ~30% of the neurons expressed ArchT lead us to estimate that we were inhibiting between 4,601–5,813 and 7,668–9,689 ArchT-expressing cells. On the other hand, if effective activation of spikes is achieved at 1.6 mW × mm −2 (threshold determined as the minimum intensity to induce spikes of striatal cells recorded in vitro ), in principle we were able to induce spikes in 30% of the neurons at least up to 0.4 (for 1 mW) and 0.8 mm (for 3 mW) from the fibre tip ( Supplementary Fig. 1g ). This distance value, together with the measured conical cross-section of 0.45 and 0.71 mm diameter at 0.4 and 0.8 mm from the fibre tip, results in a total volume experiencing 1.6 mW × mm −2 light intensity of ~0.0348 and ~0.179 mm 3 . Considering this volume and taking into account that 30% of the neurons expressed ChR2 lead us to estimate that we were activating between 930 and 4,798 ChR2-expressing cells depending on the power used. To estimate the response latency to light illumination we estimated the onset of significant firing rate decrease in the case of ArchT and increase for ChR2 after light onset, based on the neuron’s baseline firing rate peri-histogram aligned to the onset of light illumination using bins of 5 ms sliding 1 ms for ChR2 and 10 ms bins sliding 1 ms. These data analyses were conducted in Matlab with custom-written programmes (MathWorks). To estimate positive- or negative-modulated units in the postsynaptic target nuclei of either D1-ArchT or A2A-ArchT striatal manipulations ( Supplementary Fig. 4 ), we were based on 1 s baseline firing rate peri-histogram aligned to the onset of light illumination using bins of 10 ms sliding 1 bin, and only if 30 bins in the first 2 s after the onset of light were different to the baseline ( P <0.05) a unit was considered as positively or negatively modulated. Anatomical verification Three to four weeks post infection, animals were killed after completion of the behavioural tests. First, animals were anaesthetized with isofluorane, followed by intraperitoneal injection of ketamine/xylaxine (~5 mg kg −1 xylazine; 100 mg kg −1 ketamine). Animals were then perfused with saline and 4% paraformaldehyde, and brains extracted for histological analysis. Brains were kept in the same solution overnight and then transferred to saline solution. Brains were sectioned sagittally or coronally in 50 μm slices (using a Leica vibratome (VT1000S) and kept in PBS 1% solution before mounting or immunostaining treatment). After mounting and sealing of sections, one every five slices were selected to image the dorsal striatum using a confocal microscope equipped with Diodo 405 nm, Argon multi line 458-488-514 nm and a DPSS 561 nm lasers (LSM710, Zeiss; see Supplementary Fig. 1 ). Magnification ( × 40) Z stacks (50 × 50 × 50 μm; 2 μm interslice) were acquired from the upper right quadrant using a randomly positioned grid (square grid 200 μm) covering the dorsal striatum (ZEN lite software, Zeiss). These Z -stacks were imported into the stereo investigator software (MBF Bioscience) and quantification of the NeuN-positive, eYFP-positive or GFP-positive cells was done. Following this method, a total of 806/2,661 were positive for NeuN-eYFP or NeuN/GFP in ChR2 and ArchT animals ( n= 4 hemispheres; 1 RGS9L-ChR2—1 RGS9L-ArchT: 97/310, 1 D1-ChR2: 236/897, 1 D2-ChR2: 473/1454 and 1 A2A-ChR2: 50/157). To evaluate whether the RGS9L-Cre line targets the two striatal pathways we injected virus expressing protein reporters into the striatum of RGS9L-Cre animals that were generated from cross breading RGS9L-Cre animals with either D1 td-tomato or D2-eGFP . This allowed us to identify from the RGS9L-Cre -infected cell (by a DIO AAV1 virus, see above) how many of them correspond to D1-td-tomato or D2-eGFP . From three sections from three different slices in one RGS9L Cre D1 td-tomato mice we estimated that out of 347 infected cells 181 were D1 td-tomato positive (52%). On the other hand, when infecting the striatum to express td-tomato in an RGS9L-Cre D2-eGFP animal (counting the infected cells from four sections from four different slices), we estimated that 174 out of 354 infected RGS9L-Cre cells were D2-eGFP positive (49%). Software to evaluate rotations Videos from the animals in an open field were acquired using a charge-coupled device camera (DFK 31BF03) using the ICcapture software (Imaging Source) or a custom-developed software in Labview (National Instruments, Portugal) at a rate of 15 frames per second signalling in the videos of the light stimulation periods. To calculate the rostrocaudal axis, the coordinates of the head centre and the tail were determined using a custom-made software developed in Python ( https://github.com/joseaccruz/SimpleMouseTracker ). We used Matlab (MathWorks) post-hoc analyses of these coordinates to estimate rotations aligned to a one second before the light onset ( Fig. 3 , Supplementary Figs 2 and 3 ). Similarly, we used Matlab to detect the direction of the animal three frames before the light onset (the minimum number of frames to define a change in trajectory is two frames (sampling at 15 fps)—therefore, we used the minimum of three frames moving in a given trajectory to define where the body or the head was turning), to ensure that this was indeed a turning trajectory. Ipsilateral turning was plotted as positive and contralateral turning as negative ( Figs 4 and 5 , and Supplementary Figs 2 and 3 ). In these same figures for the ‘light-off’ condition we took trials using the same criteria 6 s before light onset. To further track the head rotations related to the body we vertically aligned the mouse in each frame by calculating the vertical axis of the whole animal and subtracting it for each frame (this is what we refer in the main text as subtracting the whole body axis). Once the image was vertically aligned we segmented the image, using the upper three segments to categorize the head angle and the remaining seven to determine the body angle (as depicted in Fig. 5 ). Statistics Results were represented as mean±s.e.m. and statistical significance was accepted for P <0.05. The repetition of experiments was determined above the minimum n depending on the statistical test. A non-parametric Mann–Whitney test was used for comparisons of GCaMP6s activation during baseline and turning behaviour. Paired non-parametric Wilcoxon test were performed to compare within-subject effects of the light stimulation, unless otherwise specifically stated in text. Non-parametric Kruskal–Wallis tests were used for between-subject comparisons. For statistical analyses, Matlab and Systat11 (Chicago, IL) were used. How to cite this article: Tecuapetla, F. et al. Balanced activity in basal ganglia projection pathways is critical for contraversive movements. Nat. Commun. 5:4315 doi: 10.1038/ncomms5315 (2014).